Extant diversity of bryophytes emerged from successive post-Mesozoic diversification bursts Unraveling the macroevolutionary history of bryophytes, which arose soon after the origin of land plants but exhibit substantially lower species richness than the more recently derived angiosperms, has been challenged by the scarce fossil record. Here we demonstrate that overall estimates of net species diversification are approximately half those reported in ferns and ∼ 30% those described for angiosperms. Nevertheless, statistical rate analyses on time-calibrated large-scale phylogenies reveal that mosses and liverworts underwent bursts of diversification since the mid-Mesozoic. The diversification rates further increase in specific lineages towards the Cenozoic to reach, in the most recently derived lineages, values that are comparable to those reported in angiosperms. This suggests that low diversification rates do not fully account for current patterns of bryophyte species richness, and we hypothesize that, as in gymnosperms, the low extant bryophyte species richness also results from massive extinctions. Many once-dominant land plants have either gone extinct or been reduced to an ecological role that represents just a shadow of their past importance [1] , [2] . Under the sequential replacement hypothesis [3] , [4] , the diversification of a lineage coincides with the decline of a previously dominant group. Angiosperms, which originated ∼ 200 Ma [5] , are the most recently diversifying major lineage of land plants. They underwent a rapid diversification [6] , [7] , outcompeting and outnumbering other land plants to the point of representing nearly 90% ( ca . 260,000 species) of all extant plant species [8] and defining most of the Earth’s terrestrial ecosystems since the mid-Cretaceous, ca . 100 Ma BP [9] . In contrast, bryophytes (that is, liverworts, mosses and hornworts) arose before the divergence of extant tracheophytes, soon after the colonization of land, but exhibit a comparatively lower extant diversity of ca 16,000 species [10] . Testing macroevolutionary hypotheses about bryophytes has been challenged by the scarcity of their fossil record. The earliest unambiguous macrofossil of a bryophyte dates back to the Devonian. This and other available macrofossils exhibit an overall striking similarity with extant species [11] , [12] , [13] , [14] . The similarity between ancient fossils and modern species, along with the persistence of ancestral traits such as a haploid-dominant life cycle, the dependence on water for sexual reproduction, an absence of lignified water-conducting cells, and slower rates of molecular evolution than in angiosperms [15] led to the long-held perception of bryophytes as living fossils with limited evolutionary capacities (see ref. 10 for review). One hypothesis for the comparatively lower species richness of bryophytes as compared with angiosperms is that, in line with the Sequential Replacement Hypothesis, and similar to the Cryptophytes that encompass a pool of diversity from which the ancestor of modern bryophytes and vascular plants emerged [16] , bryophytes were competitively replaced by early tracheophytes. Diversification analyses fuelled by the ever-increasing availability of molecular phylogenies and new analytical tools challenged this view but returned contrasting scenarios of bryophyte evolution. Contrary to, Shaw et al . [17] , who found that the diversification of Hypnales underwent a burst during the first 20% of their early evolutionary history, Newton et al . [18] concluded that a model of constant diversification through time was the best representation of the diversification in the pleurocarps. Wilson et al . [19] similarly concluded that the diversification of one of the major families of leafy liverworts gradually accumulated through time. Finally, Fiz-Palacios et al . [7] reported that mosses, along with ferns, opportunistically diversified in habitats newly created by angiosperms (the ‘shadow of angiosperm’ hypothesis; refs 20 , 21 ), outcompeting the more slowly speciating liverworts. Here we reconstruct and time-calibrate the phylogenies of mosses, liverworts and hornworts using the most extensive taxon and character sampling to date to demonstrate that overall estimates of net species diversification rates are approximately half the rates reported in ferns and ∼ 30% the rates described for angiosperms. Nevertheless, statistical rate analyses demonstrate that mosses and liverworts both underwent bursts of diversification from the mid-Mesozoic towards the Cenozoic to reach, in the most recently diverged lineages, net diversification rates that are comparable to those reported in ferns and angiosperms. This suggests that at least some of the major bryophyte lineages are still actively diversifying and we hypothesize that the comparatively low extant species richness in the group also results from substantial extinctions. Phylogenies Three hundred and three liverwort genera, representing 84% of the total extant generic diversity, were sequenced at eight loci from all three genomic compartments as part of a collaborative effort to reconstruct the Tree of Life. This phylogeny, together with the one previously produced for mosses [15] , was time-calibrated by relaxed molecular clock analyses, modelling the uncertainty of fossil ages used for calibration using three increasingly conservative prior distributions (see Methods). The dated phylogenies were then employed to determine net diversification rates (sensu [16] ) at different taxonomic levels, and also the tempo and amplitude of shifts in diversification rates through time. Clade age estimates The median stem age of extant moss genera (sample size=478) is 27.7±49.9, 34.2±59.8 and 41.11±68.67 Ma with calibration I, II and III, respectively. In liverworts, these values are 30.05±35 Ma, 29.7±35 Ma (sample size=303) and 37.6±42.7 Ma, and in hornworts, 32.5±43.7, 33.9±50.3 and 39.9±62.1 Ma (sample size=12; Supplementary Tables 1–3 ). These ages are older than in angiosperms (8.4±23 Ma, sample size=7,920), but lie, for mosses and liverworts, within the range reported for ferns and are much more recent than those observed in gymnosperms ( Fig. 1 , Supplementary Tables 1–7 ). The stem and crown ages of the main lineages within liverworts, mosses and hornworts are provided in Supplementary Table 8 . 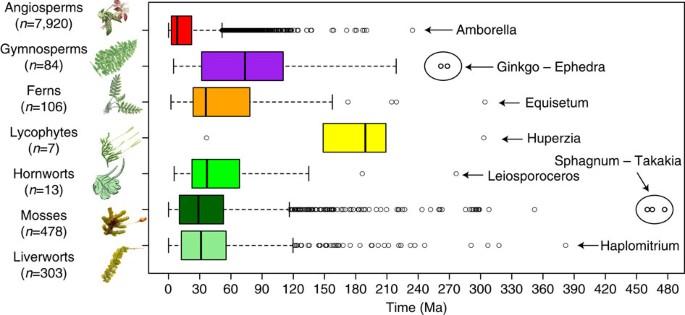Figure 1: Timing of the origin of extant genera in the major lineages of land plants. Stem ages for genera of liverworts (light green; 287 genera), mosses (dark green; 477 genera) and hornworts (bright green, 12 genera; using calibration I, seeSupplementary Tables 1–3for the results with calibrations II and III) as compared with those for lycophytes (yellow; 7 genera), ferns (orange; 106 genera), gymnosperms (purple; 84 genera) and angiosperms (red; 7920 genera) derived from ref.56. The box for each lineage represents the first and third quartiles, whiskers represent 1.5 the interquartile range, the thick bar is the median and dots are outliers genus with ages outside 1.5 the interquartile range. Figure 1: Timing of the origin of extant genera in the major lineages of land plants. Stem ages for genera of liverworts (light green; 287 genera), mosses (dark green; 477 genera) and hornworts (bright green, 12 genera; using calibration I, see Supplementary Tables 1–3 for the results with calibrations II and III) as compared with those for lycophytes (yellow; 7 genera), ferns (orange; 106 genera), gymnosperms (purple; 84 genera) and angiosperms (red; 7920 genera) derived from ref. 56 . The box for each lineage represents the first and third quartiles, whiskers represent 1.5 the interquartile range, the thick bar is the median and dots are outliers genus with ages outside 1.5 the interquartile range. Full size image Overall estimates of net species diversification rates in liverworts, mosses and hornworts are similar among the three calibration schemes. In liverworts, these rates are 0.016, 0.016 and 0.015 species per Ma with calibrations I, II and III, respectively ( Supplementary Table 8 ). In mosses, these values are 0.017, 0.017 and 0.014 and in hornworts, 0.026, 0.023 and 0.018. The net species diversification rates reported here in bryophytes are thus almost half those reported in ferns (0.028 species per Ma) and about three to four times lower than those described for angiosperms (0.09 species per Ma; Fig. 2 , Supplementary Table 8 ). High diversification rates in mosses, liverworts and hornworts were, however, observed in some of the major families such as the Ricciaceae (0.165, 0.176 and 0.139 species per Ma with calibration I, II and III, respectively), the Neckeraceae (0.086, 0.062 and 0.054) and the Anthocerotaceae (0.116, 0.110 and 0.094), and reach values that are comparable to those exhibited by individual lineages of ferns and angiosperms ( Fig. 2 , Supplementary Table 8 ). 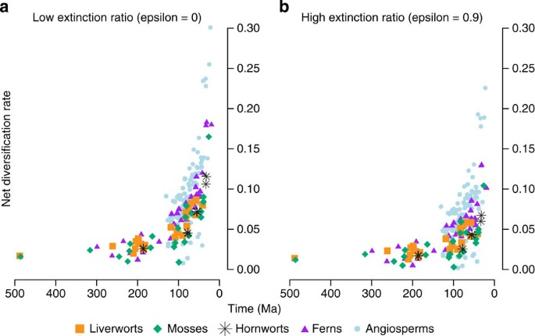Figure 2: Diversification rates among land plants. Net diversification rates (sensu22) in families and higher taxa of liverworts, mosses and hornworts resulting from the molecular dating analyses using calibration I (seeSupplementary Table 8for rates obtained with alternative calibrations). Diversification rates are shown for crown group age with low (a) and high (b) extinction risk and compared with those reported for families and higher taxa of ferns and angiosperms (see Supplementary references for literature sources). Figure 2: Diversification rates among land plants. Net diversification rates (sensu [22] ) in families and higher taxa of liverworts, mosses and hornworts resulting from the molecular dating analyses using calibration I (see Supplementary Table 8 for rates obtained with alternative calibrations). Diversification rates are shown for crown group age with low ( a ) and high ( b ) extinction risk and compared with those reported for families and higher taxa of ferns and angiosperms (see Supplementary references for literature sources). Full size image Diversification analyses A constant rate of diversification through time can be rejected in mosses and liverworts based on the results of a time-dependent diversification model. This is not the case in hornworts because of the lack of statistical power associated with the small number of genera in that group. Two significant increasing shifts in diversification rates are identified in mosses and liverworts ( Fig. 3 , Supplementary Table 9 ). The average timing of those shifts is highly congruent across the three increasingly conservative prior calibrations employed to model fossil age uncertainty ( Fig. 3 ). The average timing of the earliest diversification events in liverworts and mosses is during the mid-Jurassic and the mid-Cretaceous, respectively ( Fig. 3 , Supplementary Table 9 ). Another eight, fifteen and one increases in species diversification rate are identified by Medusa analyses in the course of the last 80 Ma in liverworts, mosses and hornworts, respectively ( Supplementary Table 10 ). 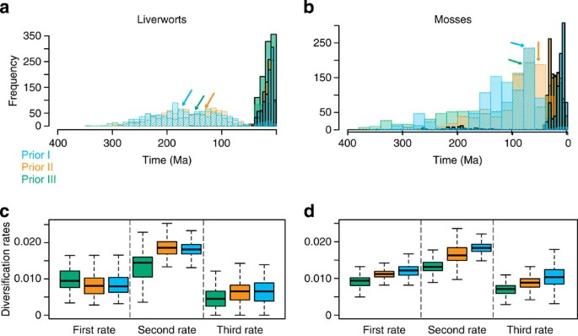Figure 3: Historical diversification shifts in bryophytes. Frequency distributions of the timing of the two significant diversification shifts (hatched bars, first shift; plain bars, second shift) in liverworts (a) and mosses (b) and genus diversification rates before the first shift (rate 1), after the first shift (rate 2) and after the second shift (rate 3;c,d) computed for 100 chronograms randomly sampled from the posterior probability distribution generated by the Beast analysis. Arrows point to the mode of the distribution. The different colours correspond to the results obtained with three increasingly conservative calibration regimes taking fossil age uncertainty into account (sky blue: calibration I; Orange: calibration II; bluish-green: calibration III; see Methods for details). The box for each calibration and rates represents the first and third quartiles, whiskers represent 1.5 the interquartile range and the thick bar is the median rates (sample size=1,000). Figure 3: Historical diversification shifts in bryophytes. Frequency distributions of the timing of the two significant diversification shifts (hatched bars, first shift; plain bars, second shift) in liverworts ( a ) and mosses ( b ) and genus diversification rates before the first shift (rate 1), after the first shift (rate 2) and after the second shift (rate 3; c , d ) computed for 100 chronograms randomly sampled from the posterior probability distribution generated by the Beast analysis. Arrows point to the mode of the distribution. The different colours correspond to the results obtained with three increasingly conservative calibration regimes taking fossil age uncertainty into account (sky blue: calibration I; Orange: calibration II; bluish-green: calibration III; see Methods for details). The box for each calibration and rates represents the first and third quartiles, whiskers represent 1.5 the interquartile range and the thick bar is the median rates (sample size=1,000). Full size image Overall estimates of net species diversification, which measure the difference between the rates of speciation and extinction weighted by the age of the lineage [22] , are clearly lower in bryophytes than in angiosperms. In line with the traditional perception of bryophytes as slow-evolving organisms, it is tempting to interpret such low diversification rates in terms of low speciation rates. Low speciation rates in bryophytes may potentially result from low levels of biotic interactions and, in particular, the absence of pollination syndromes that play a key role in angiosperm radiations (see ref. 23 for review). The high dispersal capacities of bryophytes were also assumed, in line with the extremely low levels of endemism in the group, to promote gene flow and inhibit genetic isolation, resulting in decreased opportunities for allopatric speciation [24] . Finally, strong phylogenetic niche conservatism associated with the poikilohydric condition of bryophytes may prevent them from radiating into open, disturbed environments such as the South African fynbos, where some of the most spectacular radiations of angiosperms took place [25] . Speciation and extinction rates are, however, very difficult to tease apart from phylogenies, as simulations suggested that extinction rates should not be estimated in the absence of fossil data [26] . Statistical rate analyses identified two increasing shifts in the moss and liverwort phylogenies. The average timing of those shifts was highly congruent across the three increasingly conservative prior calibrations employed to model fossil age uncertainty, confirming that increasing the width of the prior used for fossil age calibration has very little effect on the median or average age estimates but increases the confidence intervals surrounding each age estimate [27] , [28] . Liverworts exhibited an earlier shift than mosses, with an average dating back to the mid-Jurassic. This observation contrasts sharply with previous analyses of liverworts that showed a signature of declining diversification rates during the mid-Cretaceous [7] , although the difference is likely because of the use in the previous study of a higher (family) taxonomic level and lower statistical power associated with a smaller sample size. The Jurassic shift reported here in liverworts potentially points to a burst of diversification following the Permian mass extinction, during which herbaceous lycopsid and/or bryophyte-dominated terrestrial vegetation underwent an abrupt change towards an increasingly conifer-dominated vegetation [29] . In mosses, the average timing of the first shift in diversification rate dated back to the Cretaceous and adds to a growing body of evidence pointing to the ‘shadow of angiosperm’ hypothesis in a wide range of organisms as a response to an explosive increase in the structural diversity of flowering plants [30] . The second diversification rate shift observed in genus-level analyses of liverworts and mosses towards the mid-Neogene appears to be an artefact because of the fact that the sampling was limited to genera. Consequently, species diversification events were not taken into account, leading the analysis to infer a decrease in diversification rates, which corresponds to a purely methodological phenomenon known as the ‘pull of the present’ [31] , [32] . Nevertheless, analyses incorporating species richness identified another eight, fifteen and one increases in species diversification rate in the course of the last 80 Ma in liverworts, mosses and hornworts, respectively, in agreement with previous species-level phylogenetic evidence of Cenozoic diversification in selected liverwort genera [33] . Our results therefore indicate that, as opposed to the predictions of the sequential replacement hypothesis but in keeping with other lineages of ancient origin [1] , [2] , bryophytes are still actively diversifying. Consequently, net diversification rates in the most recently diverging lineages of mosses, liverworts and hornworts, such as the Hypnales (mosses), Porellales (liverworts) and Anthocerotales (hornworts), are comparable to those exhibited by individual lineages of ferns and angiosperms. This suggests that low diversification rates do not fully explain current patterns of bryophyte species richness. We therefore hypothesize that, as in gymnosperms [34] , the low extant bryophyte species richness also results from massive extinction events and highlights the need for an increased effort towards the reconstruction of their paleofloras. Taxon and molecular sampling Three hundred and three liverwort genera, representing 84% of the total extant generic diversity, were sequenced at eight loci from all three genomic compartments, including five loci of the plastid genome ( atp B, psb A, psb T, rbc L and rps 4), two genes of the mitochondrial genome ( rps 3 and nad 1) and the ribosomal 26S locus of the nuclear genome ( Supplementary Table 11 ), as part of a collaborative effort to reconstruct the Tree of Life. Six moss genera ( Sphagnum, Takakia, Andreaea, Dendrohypopterygium, Atrichum and Hookeria ) were designated as outgroups to the liverworts. In mosses, 539 of the 845 genera were sequenced for the plastid rps 4, mitochondrial nad 5 and nuclear 26S loci in the context of the Moss Tree of Life [35] . Sphagnum was employed as an outgroup. For hornworts, sequences from two plastid loci ( mat K and rbc L) and one mitochondrial locus ( nad 5) were obtained from two published studies for the 12 genera recognized to date [36] , [37] . Leiosporoceros was used as an outgroup [36] , [37] . Phylogenetic analyses The GTR+I+Γ nucleotide substitution model was selected as the best-fit model according to the BIC criterion as implemented by jModeltest [38] for each of the individual gene partitions. This model was implemented for each partition in non-parametric bootstrap analyses of 300 replicates under the ML criterion with RAxML 7.0.4 (ref. 39 ) to perform an analysis of congruence among loci before combining the data. It has been suggested that all data should be combined in phylogenetic analyses (a ‘total evidence’ approach) because different kinds of characters may help in resolving different parts of the tree and because combining data may enhance the emergence of weak, but true, signal that would be masked by noise in single-gene analyses (see ref. 40 for review). However, combining incongruent data can result in spurious clades that are supported by none of the individual partitions [41] , and therefore there is no guarantee that combing incongruent data will lead to an increase in the accuracy of the tree reconstruction. Indeed, simulation studies have shown that combining data can provide high statistical support for an incorrect species tree because of processes potentially leading to incongruence among data partition, including incomplete lineage sorting, gene duplications/extinctions (paralogy), non-neutral evolution and hybridization (see ref. 42 for review), questioning the use of a total evidence approach [43] , [44] , [45] . Incongruence was operationally defined as the presence of incompatible bipartitions found in branches supported with bootstrap proportions >95% from separate analyses of two data sets. Defining a significance level to identify incongruent bipartitions is, however, challenging and, to an extent, arbitrary, as there is no agreed upon equivalency between percentage bootstrap proportions and statistical P -values or Bayesian probabilities. Following [46] , we apply a threshold of 95%, which, while not very stringent, ensures that strongly conflicting signals between partitions are eliminated. Identification of conflicting clades between the large phylogenetic trees was aided by the use of TCT 1.5 (ref. 47 ), which outputs a list of incongruent clades. Resolution of incongruence between clades in two trees was resolved by pruning the minimum number of taxa necessary to eliminate the conflict. In liverworts, this process led to the exclusion of 16 accessions from genera, for which multiple accessions were available, so that the total number of genera was eventually not affected. In mosses, more substantial conflict was identified. For example, the Ptychomniales were the sister group to all other pleurocarpous mosses in the rps 4/ nad 5 tree, whereas, in the 26S tree, they were allied with non-pleurocarpous lineages (see ref. 35 for a complete description of the incongruence). Such conflicts resulted in a total evidence tree that was locally unresolved (see, for example, the large polytomy at the common ancestor of the Ptychomniales and Hypnales in Supplementary Fig. 1a ) and less supported ( Supplementary Fig. 1b ) than the tree obtained after exclusion of 65 genera causing incongruence among partitions. The data sets used in the present study can be obtained from http://purl.org/phylo/treebase/phylows/study/TB2:S15950?x-access-code=98d94511d8c016de8eae6f21c851826e&format=html ). Molecular dating We used an exponential uncorrelated molecular clock that implements evolutionary rate heterogeneity in BEAST 1.7.5 (ref. 48 ) to estimate divergence time. Multiple fossil constraints typically perform better than single ones [49] . The assignment of fossils to internal nodes in the phylogeny is, however, often challenged by the lack of taxonomically informative characters in fossils, an issue that is exacerbated in lineages with relatively simple morphologies such as bryophytes. Fossils such as the recently discovered moss Bryiidites utahensis [50] could not be used because they lack sufficient numbers of characters to be certain of their phylogenetic affinities. Therefore, the choice of fossils for calibration represented a trade-off between the largest amount of fossil evidence available and the extent to which the accuracy of the taxonomic position of the fossils could be determined [51] . Here 35 moss, 25 liverwort and 3 hornwort fossils, whose phylogenetic position could be unambiguously assigned, were used as calibration constraints ( Supplementary Table 12 ). Fossil evidence only provides hard minimum bounds on divergence times because the actual lineage could have been in existence long before the appearance of the calibrating fossil [52] . Using minimum bounds alone, however, provides insufficient information and can lead divergence time estimates to take arbitrarily high values, while the estimated substitution rate is driven towards very low values [52] . The use of maximum age bounds is therefore necessary; however, their definition is challenging. Choosing a young bound might indeed exclude the true divergence time, whereas choosing an old bound might return unreasonably ancient divergence time estimates [53] . Here the uncertainty of the age estimate of each fossil was modelled with a lognormal distribution under three increasingly conservative assumptions. In analysis I, the lower and upper bounds of the lognormal distribution associated to each fossil were set so as to encompass the timespan of the geological era attributed to the fossil. The lower bound for the root node was set at 475 Ma, which corresponds to the oldest non-ambiguous land plant fossil [16] . In analysis II, the lognormal distribution was centred on the fossil age estimate and the upper bound reached, for each constrained calibration node, 475 Ma. Analysis III implemented the most conservative approach possible, as the lognormal distribution employed to define the constraint at each calibration node, centred on the fossil age estimate, had a s.d. set so that its range encompasses the upper limit of the oldest inferred estimate of the origin of land plants, 815 Ma [54] . The mean and s.d. of the distributions used to model age uncertainty of each fossil are presented in Supplementary Table 12 . Four independent MCMCs were run for 200 million generations sampled every 20,000 generations. Chain stationarity and convergence were assessed by inspecting likelihood plots along each chain in TRACER [55] and by ensuring the estimate sample size values for each parameter was higher than 200. After elimination of the ‘burnin’, the log and tree posterior probability distributions were combined with LogCombiner. For graphical representation, a consensus tree was built with TreeAnnotator using the Maximum clade credibility option ( Supplementary Fig. 2 ). The median and 95% highest posterior density interval of the stem age for genera of hornworts, mosses and liverworts were compared with the stem age of genera for lycophytes (7 genera; 100%), ferns (106 genera; ±69%), gymnosperms (84 genera; 95%) and angiosperms (7,920 genera; 56%) that were retrieved from the most extensively sampled phylogeny of land plants [56] . Diversification analyses One hundred trees randomly sampled from the posterior probability distributions were employed for subsequent diversification analyses. A growing number of increasingly complex models have become available for estimating diversification rates [57] ; however, almost no comparative analysis of model performance is available yet to guide model selection [58] . Here we performed two series of complementary analyses allowing identification of shifts in diversification rate, at a global level through time on one hand, and at the level of specific lineages on the other, while taking phylogenetic and dating uncertainty into account. In the first analysis, variation in net diversification rates was modelled with a general time-dependent pure-birth model [59] with 0, 1, 2, 3 or 4 shifts in diversification through time as implemented by Ape 3.0 (ref. 60 ). Likelihood ratio tests were employed to identify the best-fit model and hence determine the optimal number of shifts. The confidence intervals of the estimated shift times were computed by profile likelihood. Sampling at the genus or higher taxonomic level leads, however, to oversampling of deep nodes and strongly biases inferences towards downturns, a purely methodological phenomenon known as the ‘pull of the present’ [31] , [32] . A second series of diversification analyses that takes species richness in each genus into account ( Supplementary Tables 11 and 13 ) and identifies breakpoints in diversification rates in specific lineages was therefore performed with a pure-birth model as implemented by MEDUSA 0.93.4-30 (ref. 61 ). In the current context of taxonomic changes fuelled by the ever-increasing availability of molecular data, available species numbers must be considered as a trade-off between two general trends. The first is that molecular evidence has led to an increase in the description of new species in groups with reduced or overlapping morphologies. The converse trend is that recent global taxonomic work points to the need for extensive synonymizations, as hundreds of ‘geographical species’ were described based in large part on the assumption that populations from distant regions must represent species distinct from familiar European taxa [62] . Although the species number used here must be considered with caution, as they represent rough estimates that are likely to be modified as taxonomic evidence accumulates, they provide reasonable proxies for comparisons between small and large genera, and can be informative with regards to global diversification patterns. Net species diversification rates were computed for stem and crown groups in the main lineages of hornworts, mosses and liverworts following equations 6 and 7 from ref. 22 using the bd.ms() function in the R package geiger 1.99-3.1 (ref. 63 ) and compared with estimates from the literature for ferns and angiosperms (see Supplementary Table 8 for details). A relative extinction rate ( ɛ ) defined as ɛ = μ / λ where μ and λ are the absolute extinction and speciation rates, respectively, was used to contrast two extreme scenarios, with ɛ =0 representing no extinction and ɛ =0.9 representing a relatively high extinction rate. How to cite this article: Laenen, B. et al . Extant diversity of bryophytes emerged from successive post-Mesozoic diversification bursts. Nat. Commun. 5:5134 doi: 10.1038/ncomms6134 (2014).